Discovery of gigantic molecular nanostructures using a flow reaction array as a search engine The discovery of gigantic molecular nanostructures like coordination and polyoxometalate clusters is extremely time-consuming since a vast combinatorial space needs to be searched, and even a systematic and exhaustive exploration of the available synthetic parameters relies on a great deal of serendipity. Here we present a synthetic methodology that combines a flow reaction array and algorithmic control to give a chemical ‘real-space’ search engine leading to the discovery and isolation of a range of new molecular nanoclusters based on [Mo 2 O 2 S 2 ] 2+ -based building blocks with either fourfold (C 4 ) or fivefold (C 5 ) symmetry templates and linkers. This engine leads us to isolate six new nanoscale cluster compounds: 1 , {Mo 10 (C 5 )}; 2 , {Mo 14 (C 4 ) 4 (C 5 ) 2 }; 3 , {Mo 60 (C 4 ) 10 }; 4 , {Mo 48 (C 4 ) 6 }; 5 , {Mo 34 (C 4 ) 4 }; 6 , {Mo 18 (C 4 ) 9 }; in only 200 automated experiments from a parameter space spanning ~5 million possible combinations. Understanding and controlling the self-assembly of complex inorganic molecules is a non-trivial problem often relying on serendipity rather than a systematic or predictive search [1] , [2] . Such unpredictability is especially true for kinetically labile systems such as in coordination cluster chemistry, where the numerous coordination modes and configurations open to transition metals meaning the time required to explore the experimental parameter space would be prohibitive. Yet the ability to design, predict or at least systematically discover new clusters could be transformative due to their many potential applications in nanotechnology [3] , magnetism [4] and redox active [5] , water oxidation [6] . These problems are exacerbated in polyoxometalate chemistry, where nanoscale clusters with over 350 metal ions in a single molecule have been discovered [7] , [8] , [9] . Polyoxometalate cluster science is an interesting area since the starting reagents are deceptively simple involving the condensation of ‘monomeric’ metal oxo units for example, {Mo x } (where M is typically V, Mo, W, Nb in high oxidation state) into ‘polymers’ of these units via shared oxo-ligands. Indeed the very large number of clusters that can be generated represents a vast combinatorial problem, and it is currently impossible to explore the available search space in any sensible way using standard ‘beaker’ or one-pot experiments due to the static constraint of the reaction variables (requiring a vast number of experiments to cover all the combinations and permutations) [9] , [10] . As such the need for a configurable and repeatable methodology for the discovery and reproducibility of novel transition metal cluster compounds, of which POM clusters are a fundamental example, is paramount. In this regard, we have recently proposed that configurable reactors to automate the continuous variation of the reaction variables for example, reagent concentration, combination, process conditions and networking of reactor systems could transform our ability to both discover and scale-up molecular nano-inorganic clusters [11] , [12] , [13] . Herein, we describe the computer control of a multi-input continuous flow reactor system to explore the search space like a real-space ‘synthetic chemistry search engine’ (by ‘real-space’ we mean that the search is done experimentally rather than an in-silico simulation or literature-based predictive system) exploring the self-assembly of clusters employing well-defined building units, organic templates, plus labile and geometrically diverse building units to discover novel polyoxothiometalates (POTMs). The key advantages of this system include rapid homogeneous mixing and also fast processing/reproduction of reaction mixtures to discover new chemical architectures in an automated manner, avoiding laborious and time-consuming conventional one-pot reactions, as shown by the discovery of the giant macrocylic {Mo 96 } [12] . Further, the use of new templates, as hinted at in previous work, reveals the potential of the chemical space. This is because different organic templates can be used to influence the self-condensation process of dithiomolybdate moieties giving an unpredictable and large parameter space to be searched [14] , [15] ; indeed Cadot and co-workers [16] have reported that flexible organic ligands have a massive templating influence on the self-condensation of dithiomolybdate [Mo 2 O 2 S 2 ] 2+ , but little work has involved the use of rigid, planar organic ligands. In addition, we reason that it should be possible to introduce both the organic templates and virtual polyoxometalate clusters (addenda anions) concurrently to increase the geometrical complexity of the components explored by the reaction array and investigate gradual changes in reaction composition. Herein we purposely choose a library of starting materials so we can explore and develop our configurable reactor ‘search engine’ for instance by varying the geometry of the organic templates, addenda anions and pH influence the self-condensation of [Mo 2 O 2 S 2 ] 2+ -building units which taken together represents a vast combinatorial problem [17] . As such, by using a flow approach to explore new reaction spaces, we demonstrate that it is possible to automate the search and investigate many different parameters for example, volume/concentration, reagent combination, temperature and so on. This is because the parameters can be varied in a continuous stream, rather than in discrete batches as in the traditional ‘one-pot’ synthesis. 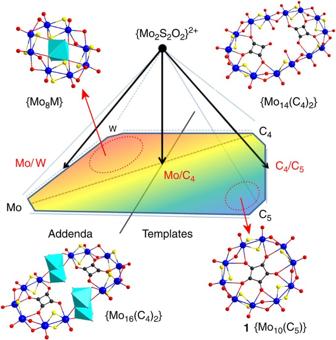Figure 1: Exploring the reaction space with search engine. Individual experiments fixed the concentrations of three components while altering the concentration of two other components. {Mo2} is an essential component, regardless of its selection from either squarate (C4) or croconate (C5), which acts as organic template components, and selects from either Mo or W that acts as addenda anion component. Colour code: Mo, blue spheres and cyan polyhedra; S, yellow spheres; C, black spheres; O, red spheres; Mo6template, sky blue polyhedron (M: Mo or W). This means that several changing parameters can be explored at the same time, potentially covering a bigger search space than is possible by the linear combination of variables, as is done in the batch format (see Supplementary Table 1 for flow algorithm). Here we exemplify this approach in the discovery of six new POTM clusters and also reliably reproduce four previously reported compounds (which themselves exist in a vast parameter space and their reproducible synthesis had been extremely challenging, if not impossible, in some cases) [12] , [18] , [19] . Furthermore, this search engine approach also defines a new method by which mechanistic details may be probed helping understand the variables important for cluster formation. In this respect, it is worth noting that Müller et al. [20] have been exceptionally successful in using one-pot reactions for the synthesis of a series of high nuclearity polyoxomolybdates including the spherical {Mo 132 } (ref. 20 ), wheel-shaped {Mo 154 } (ref. 21 ) and blue lemon {Mo 368 } (ref. 22 ), but it is entirely conceivable that a massive library of other possible clusters maybe available but are difficult to or impossible to isolate under single-pot conditions. This is because these reduced Mo-POMs contain a range of dynamic combinatorial virtual building blocks (VBBs—first realized and discussed by Müller et al. ) [22] that could be combined in a number of ways giving a virtual library of structures arising from different hypothetical combinations of these building blocks. For example, in the case of the spherical {Mo 132 } cluster species, the building blocks can be thought to be based on the pentagonal {Mo(Mo 5 )} and dimeric {Mo 2 } units, or as a single {Mo 8 } building block. To date, no one has isolated any such molybdate or tungstate VBBs independently of such ball- or wheel-shaped clusters presumably due to the high lability of such species [23] , [24] . However, we hypothesize that the [Mo 2 O 2 S 2 ] 2+ thiometalate cation may be used to help trap these VBBs in solution to form novel clusters, as recently shown in squarate (C 4 O 4 )-templated POTMs (C 4 -POTMs) which can either trap [Mo 2 O 7 ] 2− to form a ‘Möbius strip’ topology [18] , or [Mo 5 O 18 ] 6− to generate high nuclearity clusters [19] . Following our previous work, we are motivated to trap exotic VBBs, such as the pentagonal unit {Mo(Mo 5 )}, to construct a novel series of clusters by systematically exploring reaction arrays and chemical compositions of reactions. Selection of building blocks For each set of reactions, a known starting point in the synthetic parameter space was sought, typically this was based on previously reported compounds which have been structurally characterized. By using known compounds with a given set of structurally characterized building blocks, we can use this as an indication of available building blocks under the conditions previously specified. As such, we reasoned it would be interesting to use such set points to vary the concentrations of certain key components to expand and explore the combinatorial space around the initial established composition. For instance, by varying the ratio of dithiomolybdate [Mo 2 O 2 S 2 ] 2+ versus organic templates (squarate, C 4 O 4 2− and croconate, C 5 O 5 2− anions) and versus addenda (molybdate, Na 2 MoO 4 and tungstate, Na 2 WO 4 ) we generated five-component sequences of systematic screenings, see Fig. 1 . Figure 1: Exploring the reaction space with search engine. Individual experiments fixed the concentrations of three components while altering the concentration of two other components. {Mo 2 } is an essential component, regardless of its selection from either squarate (C 4 ) or croconate (C 5 ), which acts as organic template components, and selects from either Mo or W that acts as addenda anion component. Colour code: Mo, blue spheres and cyan polyhedra; S, yellow spheres; C, black spheres; O, red spheres; Mo 6 template, sky blue polyhedron (M: Mo or W). 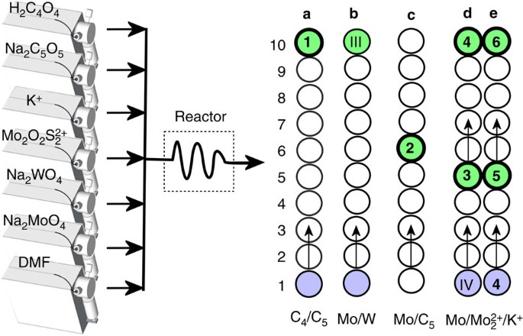Figure 2: Diagram of the search engine system. The exploration of the combinatorial space was based on running five different sets of experiments (a–e), using a common batch of stock solutions of the building blocks. The search approach in the experiments was based on changing ratio between C4and C5(a); between Mo and W (b); between Mo and C5(c); finally, a three-component variation between Mo, {Mo2}2+and potassium source/medium (dande) was also used. Full size image Autonomous screening of reaction compositions Here, the search engine comprises a flow system array [12] that rapidly generates multiple chemical reactions in a systematic and automated fashion controlled algorithmically (see Supplementary Table 2 ). In this sequence-controlled algorithm, five different sets of experiments using a common batch of stock solutions were performed. At the start of the experiments ( t =0), the total flow rate is set at 4 ml min −1 for all the inputs, and a target volume of 10 ml per reaction is set, and this reaction occurs within a tubular reactor. We constructed five separate parallel sets of principal reactions to be performed ( Fig. 2 ) within each principal reaction where a subset of the 10 reactions were varied systematically with respect to at least two of the key components. Subsequent reactions saw more key components varied with respect to each other, up to four or five separate parameters per reaction set. Each individual reaction had exactly the same total volume as every other reaction. In each set of reactions, all reagent-mixing ratios were programmed by the computer control system using our chemical-search algorithm using the variables defined above, and then the experiments were autonomously undertaken using prepared stock solutions of reagents. The flow set up used seven programmable syringe pumps controlled by a LabVIEW-based PC interface. Six reagent stock solutions were connected to the assigned inlets for 5-ml syringe pumps and one more 12.5-ml syringe pump was used to deliver an ‘air plug’ between reactions. Figure 2: Diagram of the search engine system. The exploration of the combinatorial space was based on running five different sets of experiments ( a – e ), using a common batch of stock solutions of the building blocks. The search approach in the experiments was based on changing ratio between C 4 and C 5 ( a ); between Mo and W ( b ); between Mo and C 5 ( c ); finally, a three-component variation between Mo, {Mo 2 } 2+ and potassium source/medium ( d and e ) was also used. Full size image Key factors determining the self-condensation of POTMs To help design the experiments, we first explored the influence of certain key components in the self-condensation of POTMs, primarily organic templates and addenda anions. The first parameter to be studied was the influence of organic templates. The starting composition for this was the known {Mo 14 (C 4 ) 2 } ring [18] , composed of two squarate anions (one rotated 45° to the other) encapsulated inside a 14-member molybdenum ring. We reasoned that a combination of another rigid organic template may well lead to the discovery of new structures, and this lead to six new compounds as listed in Table 1 . Our initial exploration started by varying the ratio of the fourfold symmetric squarate to fivefold symmetric croconate anions. From our screenings, the only combination that gave rise to a new product was entry ‘a10’, see Supplementary Table 2 . X-ray crystallographic analysis of the crystals produced from the mother liquor revealed a thiomolybdate ring perfectly coordinated to a single croconate anion template {Mo 10 (C 5 )}=[N(CH 3 ) 4 ]K[(Mo 2 O 2 S 2 ) 5 (OH) 10 (C 5 O 5 )] · 17 H 2 O ( 1 ), see Fig. 1 and Supplementary Fig. 2 , and this showed rather remarkably that the symmetry of the fivefold croconate anion could be mapped onto the ring structure perfectly. Next, we probed the influence of addenda anions in the form of MoO 4 2− and WO 4 2− . Here the starting point for this set of reactions was {Mo 16 (C 4 ) 2 }, a slightly larger ring than {Mo 14 (C 4 ) 2 }, but where the two squarate anions inside the ring are orientated parallel to each other. When the addenda (‘b’ entries, see Supplementary Table 2 ) were used in the pH rises up to 5.5–7 range, simple {Mo V 8 (M VI )} clusters (M=Mo and W) appeared as the sole products [25] , [26] , [27] , [28] . Table 1 Summary of anion formulae for each of the clusters in this work. Full size table Fine tuning reaction parameters The initial results gave us a great deal of new understanding as to which parameters had the greatest influence on cluster nuclearity and shape. We then aimed to incorporate the croconate into an even more complex structure; this was achieved by exploring the ratio of croconate versus molybdate in the presence of squarate template and thiomolybdate. Under these conditions, entry ‘c6’ produced a chiral co-crystallizing compound {Mo 14 (C 4 ) 4 (C 5 ) 2 }=K 10 [(Mo 2 O 2 S 2 )(H 2 O) 2 (C 5 O 5 ) 2 ][Mo 12 O 36 (C 4 O 4 ) 4 ] · 14 H 2 O ( 2 ) within the space group P 2 1 , featuring a {Mo VI 12 (C 4 ) 4 } squarate cage [29] and a novel thiomolybdate-croconate fragment, see Fig. 3a . Interestingly, no C 5 -templated wheel was found when adding C 4 component to the chemical mixture, contrary to our expectations. It became rapidly apparent that inclusion of both croconate and tungstate components diverted reaction pathways into structurally small, fast kinetic wheel products ( 1 and {Mo 8 (W)}), thus we omitted them from future experiments. 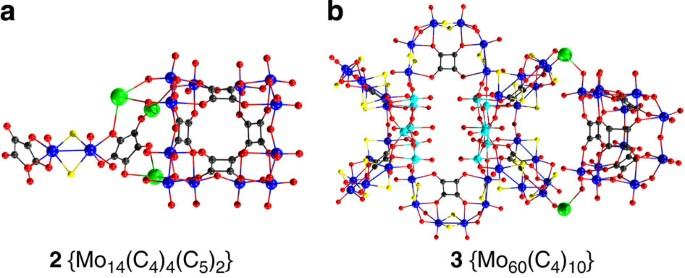Figure 3: Co-crystallizing POTM-POMs discovered during screening. (a) X-ray crystal structure of2{Mo14(C4)4(C5)2} and (b)3{Mo60(C4)10}. Colour code: Mo, blue spheres; S, yellow spheres; C, black spheres; O, red spheres; K, green sphere; {Mo(Mo5)} pentagonal unit, cyan spheres. Figure 3: Co-crystallizing POTM-POMs discovered during screening. ( a ) X-ray crystal structure of 2 {Mo 14 (C 4 ) 4 (C 5 ) 2 } and ( b ) 3 {Mo 60 (C 4 ) 10 }. Colour code: Mo, blue spheres; S, yellow spheres; C, black spheres; O, red spheres; K, green sphere; {Mo(Mo 5 )} pentagonal unit, cyan spheres. Full size image The starting point for the next set of reactions was the giant {Mo 96 (C 4 ) 12 } cluster, which was highlighted during flow-based experiments in our key previous report [12] , and extensively studied in [Mo 5 O 18 ]-trapping studies [19] . The components to be varied were thiomolybdate versus K 2 CO 3 . Entry ‘d5’ yielded structure {Mo 60 (C 4 ) 10 }=[N(CH 3 ) 4 ] 4 K 18 [((Mo 2 O 2 S 2 ) 3 (OH) 4 (C 4 O 4 )) 6 (OH) 2 (Mo 6 O 21 (H 2 O)) 2 ] [Mo 12 O 36 (C 4 O 4 ) 4 ] · 79 H 2 O ( 3 ), comprising the same squarate {Mo 12 (C 4 ) 4 } cage in 2 plus a novel [Mo 2 O 2 S 2 ]-based molecular architecture namely {Mo 48 (C 4 ) 6 }={Mo 48 }, see Fig. 3b . The appearance of a new {Mo 48 } cluster within a novel co-crystallizing structure spurred us on to synthesize {Mo 48 } by itself. Thus, we took the above conditions but changed the molybdate constant to a variable. The naked {Mo 48 (C 4 ) 6 }=[N(CH 3 ) 4 ] 3 K 11.5 Na 0.5 I[((Mo 2 O 2 S 2 ) 3 (OH) 4 (C 4 O 4 )) 6 (OH) 2 (Mo 6 O 21 (H 2 O)) 2 ] · 90 H 2 O ( 4 ) cluster was isolated from the conditions listed in entry ‘d10’, see Fig. 4a . The {Mo 48 } cluster represented the class of target structure we initially set out to discover within the VBB possibilities, thus we used these conditions to search for novel cluster re-arrangements. Having screened a large reagent space we decided to vary five key components, molybdate, thiomolybdate, K 2 CO 3 , squarate (C 4 O 4 2− ), plus we swapped KCl for KAc as potassium source. Entry ‘e5’ gave rise to a novel smaller cluster {Mo 34 (C 4 ) 4 }={Mo 34 }=K 14 [((Mo 2 O 2 S 2 ) 3 (OH) 4 (C 4 O 4 )) 4 (Mo 5 O 18 (CH 3 COO)) 2 ]· 52 H 2 O ( 5 ) containing one lacuna pentagonal {Mo 5 }-containing cluster, at a higher pH value of 4.6, see Fig. 4b . Finally, to probe solvent effects we investigated a water:DMF co-solvent mixture. Using the composition for {Mo 34 } as a starting point by adding KCl as potassium source and DMF, we yielded a smaller {Mo 18 (C 4 ) 9 }={Mo 18 }=[N(CH 3 ) 4 ] 4 K 8 [((Mo 2 O 2 S 2 ) 3 (OH) 4 (C 4 O 4 )) 3 (C 4 O 4 ) 6 (N(CH 3 ) 2 CHO) 3 ] · 30 H 2 O ( 6 ) cluster than 5 at pH 3.2, see Fig. 4c . 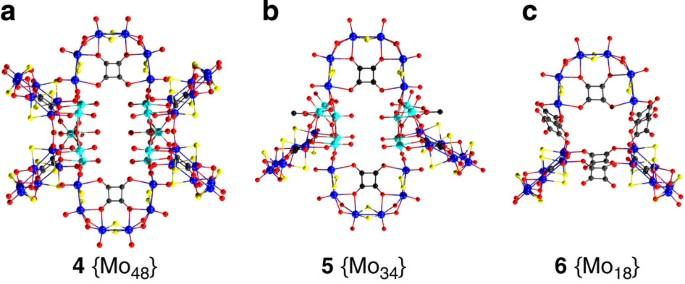Figure 4: The C4-POTMs discovered during screening. X-ray crystal structures of (a)4{Mo48} 24.5 × 23.0 Å, (b)5{Mo34} 22.5 × 23.7 Å and (c)6{Mo18} 17.1 × 17.2 Å. Colour code: Mo, blue spheres; S, yellow spheres; C, black spheres; O, red spheres; K, green sphere; {Mo(Mo5)} pentagonal/{Mo(Mo4)} lacunary pentagonal unit, cyan spheres. Figure 4: The C 4 -POTMs discovered during screening. X-ray crystal structures of ( a ) 4 {Mo 48 } 24.5 × 23.0 Å, ( b ) 5 {Mo 34 } 22.5 × 23.7 Å and ( c ) 6 {Mo 18 } 17.1 × 17.2 Å. Colour code: Mo, blue spheres; S, yellow spheres; C, black spheres; O, red spheres; K, green sphere; {Mo(Mo 5 )} pentagonal/{Mo(Mo 4 )} lacunary pentagonal unit, cyan spheres. Full size image One of the key aspects of the system is that we are able to exploit the unpredictable nature of inorganic cluster self-assembly processes in general using an algorithmic reaction engineering paradigm. This means that we are able to go beyond the linear combination of components leading to a predefined library of outcomes since the entire process is not predictable, say compared with some combinatorial synthesis. For instance, our attempt at inclusion of a second organic template was an important parameter to probe. However, as became readily apparent, the fivefold croconate template proved to be a perfect template, too perfect in fact. This is because croconate anion is the ideal size to template the self-condensation of five thiomolybdate-building blocks to create a deca-membered ring, 1 {Mo 10 (C 5 )} (see Fig. 1 ), the crystal structure possesses a high symmetry, approximately D 5 h . The five [Mo 2 O 2 S 2 ] 2+ units are connected via hydroxyl anion bridges to form the ring; each oxygen atom of the croconate anion has bifurcated interactions (ranging from 2.44(8) to 2.86(0) Å) to two Mo V atoms from separate [Mo 2 O 2 S 2 ] 2+ -building blocks. Interestingly, each [Mo 2 O 2 S 2 ] 2+ unit is parallel to each conjugated C–C bond and the bridging hydroxo groups are in the direction of the oxygen atoms of the croconate anion ( Supplementary Fig. 2 ). Comparing the template effect present in {Mo 14 (C 4 ) 2 } (ref. 18 ) and 1 , the polyoxothiometalate rings differ in the nuclearity and shape of the cluster, from an ellipsoid to a circular ring in 1 ( Fig. 1 and Supplementary Fig. 3 ). We propose that the geometry of the squarate anion inhibits the formation of a circular ring because of the high steric strain such a ring would be under. Comparatively, the length of each {[Mo 2 O 2 S 2 ](OH) 2 } unit combined with the pentagonal geometry of the C 5 O 5 2− template overcomes any steric hindrance resulting in the formation of a perfect circular ring. The downside of the perfect match between croconate and thiomolybdate-building blocks is that it is extremely hard to incorporate this organic template into larger POTM clusters, whereas it was much easier to utilize squarate as an organic template allowing more divergent structures from the ‘imperfect’ half ring architectures. By exploring the solution behaviour of the molecule using mass spectrometry, compound 1 , the cluster is stable in solution with the peaks at m/z =875.3 and 1,824.8 attributed to −2 and −1 charged molecular ion peaks ( Supplementary Fig. 4 , Supplementary Table 3 ). Another false avenue was the attempted inclusion of tungstate addenda; we regard this situation as an example of template competition and also in the pH range studied as the MO 4 2− addenda serve as better templates than C 4 O 4 2− , leading to the formation of {Mo 8 W} [25] and {Mo 8 Mo} clusters [27] . The nanosized ‘butterfly-like’ cluster 4 {Mo 48 } ( Fig. 4a ) contains two different types of building blocks: two {Mo(Mo 5 )} pentagonal-building blocks and six neutral [(Mo 2 O 2 S 2 ) 3 (OH) 4 (C 4 O 4 )]≡{Mo 6 (C 4 )} half-circles self-condensed about a central squarate anion. Although the size of the croconate anion allows a perfect fit of five [(Mo 2 O 2 S 2 )(OH) 2 ] units around its circumference, the squarate anion cannot coordinate four [(Mo 2 O 2 S 2 )(OH) 2 ] units around itself to form a closed ring as the steric strain would be prohibitive. Instead, squarate coordinates only three [Mo 2 O 2 S 2 ] 2+ units to form a semi-circular {Mo 6 (C 4 )} unit with electrophilic attachment points, ready to trap other species, be it pentagonal units or organic anions. Although the {Mo 6 (C 4 )}-building block is neutral, the two-edge Mo V atoms are unsaturated and can act as electrophilic groups. At low pH ( ca . 2–3), the negatively charged [Mo VI 6 O 21 (H 2 O)] 6− pentagonal-building block serves as a nucleophilic group attracting a total of four electrophilic Mo V centres from two {Mo 6 (C 4 )}-building blocks, which attach to the pentagonal unit via Mo-O bonds (Mo-O=2.04(4)–2.35(5) Å). The {Mo 6 (C 4 )} units sit on the same face of the pentagonal unit with ca . 90° opening between them to form the ‘wings’ of the butterfly, see Fig. 5 . Two more {Mo 6 (C 4 )}-building blocks, placed top and bottom perpendicular to the initial {Mo 6 (C 4 )} units, bridge the two pentagonal ‘wing’ units to form the complete {Mo 48 } cluster. It is worth mentioning that on each side, the ‘wings’ of the cluster are connected and fixed by OH − via Mo-OH bonds (2.07(5)–2.13(2) Å). According to Bond Valence Sum (BVS), the molybdenum centres in the pentagonal unit maintain a +VI oxidation state, while the thiometalate Mo have +V valence state. It is worth noting that this [Mo VI 6 O 21 (H 2 O)] 6− is slightly different from the previously reported one [8] , because one Mo VI is five coordinate and shows a square-based pyramidal geometry, while in the previously reported pentagonal unit, all the Mo VI atoms have octahedral geometry ( Supplementary Fig. 5 ). The reason for the difference is that the five coordinate Mo VI atom tilts upward, causing steric hindrance thus preventing coordination of a sixth oxygen atom. Additionally, the central Mo VI atom of the pentagonal unit is coordinated by water molecules ( Supplementary Fig. 5c ) and the clusters pack along c axis in order ( Supplementary Fig. 6 ). It is interesting to find that at a higher pH value, the lacuna pentagonal-building block {Mo 5 }={Mo 5 O 18 (CH 3 COO)} formed instead of a full pentagonal unit {Mo(Mo) 5 }, thus only four {(Mo 2 O 2 S 2 ) 3 (OH) 4 (C 4 O 4 )} subunits can link onto two {Mo 5 } units leading to an ‘incomplete butterfly’ architecture 5 {Mo 34 } ( Supplementary Fig. 7 ). There is disorder in the acetate molecule coordinating to the {Mo 5 } unit via Mo-O bonds, ranging from 2.16 to 2.28 Å. 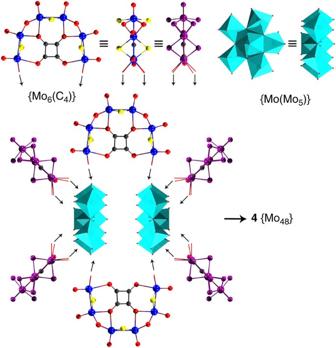Figure 5: Plausible representation of formation of4{Mo48}. Two building blocks {Mo6(C4)} (purple) coordinate, at 90° relative to each other, to the pentagonal unit via Mo-O bonds to form the ‘wings of {Mo48}. The two wings are bridged by two further {Mo6(C4)} units to construct {Mo48}4. (Pentagonal unit {Mo(Mo5)}: cyan polyhedra; ball-and-stick representation for C: black; MoV: blue; S: yellow; O: red.)Supplementary Movie 1shows how the cluster compound is constructed. Figure 5: Plausible representation of formation of 4 {Mo 48 }. Two building blocks {Mo 6 (C 4 )} (purple) coordinate, at 90° relative to each other, to the pentagonal unit via Mo-O bonds to form the ‘wings of {Mo 48 }. The two wings are bridged by two further {Mo 6 (C 4 )} units to construct {Mo 48 } 4 . (Pentagonal unit {Mo(Mo 5 )}: cyan polyhedra; ball-and-stick representation for C: black; Mo V : blue; S: yellow; O: red.) Supplementary Movie 1 shows how the cluster compound is constructed. Full size image The mass spectrum of 3 {Mo 60 } proves that the two clusters separate in solution and the main peak represents the main butterfly cluster {Mo 48 } that retains its structural integrity ( m/z =1,719.4, 2,108.7, 2,163.7), but only partial fragments of the cage can be detected ( m/z =1,809.9, 2,333.8) ( Supplementary Fig. 8 and Supplementary Table 4 ). As for compound 4 in a mixture of deionized water and acetonitrile (5:95%) shows peaks at m/z =1,640.6 and 1,715.6 corresponding to the presence of {((Mo 2 O 2 S 2 ) 3 (OH) 4 (C 4 O 4 )) 6 (OH) 2 (Mo 6 O 21 (H 2 O)) 2 } 14− , while the cluster fragments are also exhibited, mainly {((Mo 2 O 2 S 2 ) 8 (OH) 11 (C 4 O 4 ) 2 )(Mo 6 O 21 (H 2 O))} 5− at m/z =1,246.4 and 1,343.1 ( Supplementary Fig. 9 and Supplementary Table 5 ). The POTM cluster 6 {Mo 18 } forms without trapping any pentagonal molybdate-building blocks. According to the X-ray crystallography, the compound crystallizes in the P 2/ c space group with approximately C 2 v symmetry ( Supplementary Fig. 10 ). Two {(Mo 2 O 2 S 2 ) 3 (OH) 4 (C 4 O 4 )} units are connected by two squarate anions via Mo-O bonds (Mo-O=2.12(4)–2.16(1) Å) to form the {((Mo 2 O 2 S 2 ) 3 (OH) 4 (C 4 O 4 )) 2 (C 4 O 4 ) 2 } bottom half. To complete the {Mo 18 } cluster, four additional squarate anions coordinate onto the four unsaturated Mo V atoms facilitating the capping by a final {(Mo 2 O 2 S 2 ) 3 (OH) 4 (C 4 O 4 )} unit, placed perpendicular to the initial two {(Mo 2 O 2 S 2 ) 3 (OH) 4 (C 4 O 4 )} units. Two interesting compounds comprising co-crystallizing molecules emerged during this study, both feature a {Mo 12 } cage which was first reported by Zubieta [29] with potassium cations bridging the separate clusters. The {Mo 12 } cage is the product of an excess of squarate anions and molybdate in solution and consists of four edge-sharing {Mo 3 O 14 } coordinated polyhedra connected to each other via corner sharing and fixed in place by four squarate ligands; the inner cavity possesses a diameter of ca . 2.5 Å. The first example is the only structure in this study to feature both squarate and croconate template anions together in the same crystal structure, {Mo 14 (C 4 ) 4 (C 5 ) 2 }. The fragment incorporating the croconate anion seems to be the result of the trapping of a single unit of [Mo 2 O 2 S 2 ] 2+ between two C 5 O 5 2− anions giving a [(Mo 2 O 2 S 2 )(H 2 O) 2 (C 5 O 5 ) 2 ] 2− motif. This is quite unusual as other syntheses involving croconate that yield any product produced only wheel 1 {Mo 10 (C 5 )}. The cluster 2 is another example of spontaneous resolution in the absence of any chiral source [30] . The chirality originates from the helical packing of compound 2 along the c axis with {Mo 12 } cages located in the grooves of the helix ( Supplementary Fig. 11 ). The second co-crystallizing example was produced when the system had an excess of C 4 O 4 2− and molybdate giving rise to 3 {Mo 60 }. This compound comprises the {Mo 48 } cluster, co-crystallizing with a {Mo 12 } cage bridged by a two potassium cations. The majority of the clusters discovered here are comprised mainly of the {Mo 6 (C 4 )} squarate-POTM-based building block, furthermore, we observed two different VBBs, the pentagonal [Mo 6 O 21 (H 2 O)] 6− and the lacunary {Mo 5 }, plus kinetic fragments, {Mo 2 (C 5 ) 2 }. As it is well documented, aqueous solutions of molybdate are unique in that they allow the generation of a huge variety of virtual building block libraries, which is the reason why two or even more building blocks often appear in one compound. However, in our case, the {Mo 6 (C 4 )}-building block can trap different building blocks separately, which provides profound proof for the existence of the building blocks. The pH value is an important factor for influencing whether the complete pentagonal or the lacunary pentagonal unit will form: at low pH 2–3, it is more likely that the pentagonal unit [Mo 6 O 21 (H 2 O)] 6− forms, while when pH is increased to 4.6, the lacunary pentagonal unit [Mo 5 O 18 (CH 3 COO)] forms. The {Mo 6 (C 4 )}-building block can exist in a wide pH range 2–5 and it exists in several compounds. However, it is not always the case that large aggregates of thiometalates can form. If the template is too perfect for the self-condensation of [Mo 2 O 2 S 2 ] 2+ , it is hard to get large aggregates of POTMs. Similarly, the addenda tungstate is not suitable to extend the semicircle virtual building block {Mo 6 C 4 } to form large clusters but the small aggregates {Mo 8 W}. In conclusion, we used an automated flow system to explore the self-condensation of [Mo 2 O 2 S 2 ] 2+ under different templates and addenda environments using a well-defined algorithm for the combination of the components. The perfect fivefold symmetric template C 5 O 5 2− prohibits the expansion of larger POTMs; however, the fourfold symmetric squarate template induces three [Mo 2 O 2 S 2 ] 2+ units to form the semi-circular ring {Mo 6 C 4 } with reactive ends, which can be extended by either the polyoxomolybdate-building blocks or squarate anions to form larger clusters. Using MoO 4 2− ions as addenda units plays a positive role in expansion of POTMs, but that is not the case for the WO 4 2− . Not only does the automated system allow us to dramatically speed up our search of the [Mo 2 O 2 S 2 ]-based parameter space, it also has the potential for us to design experiments to probe how the large clusters form under certain conditions. The above results will be useful for synthetic chemists for future experiment design, as well as developing better search algorithms, using feedback control to move more exhaustively through the search space, especially when the combinatorial space is non-linear and discovery rather than prediction is the name of the game. Materials and chemicals All chemicals were of analytical reagent grade purchased from Sigma Aldrich and Alfa Aesar chemical companies and used as supplied without further purification. The standard stock solutions of each reagent were prepared using standard practices and volumetric glassware. All solutions were prepared with deionized water and stored in glassware after preparation. The [Mo 2 O 2 S 2 ] 2+ solution (containing (CH 3 ) 4 N + and I − ions) was prepared according to the literature procedure [31] and it was always stored in Ar till used. The reagent stock solutions were prepared as follow: Na 2 MoO 4 ·2 H 2 O (4.84 g, 20 mmol) was dissolved in water and made up to 100 ml to give a 0.2-M molybdenum stock solution. Squaric acid C 4 O 4 H 2 (1.93 g, 16.9 mmol) was dissolved in deionized water and made up to 100 ml to give a 0.17-M squaric acid stock solution. Croconate sodium salt C 5 O 5 Na 2 (1.86 g, 10 mmol) was dissolved in 100 ml deionized water to give a 0.1-M croconic sodium stock solution. K 2 CO 3 (1.38 g, 35 mmol) was dissolved in deionized water and made up to 100 ml to give a 0.35-M potassium carbonate stock solution. Na 2 WO 4 · 2 H 2 O (16.5 g, 50 mmol) was dissolved in water and made up to 100 ml to give a 0.5-M molybdenum stock solution. KCl (3.7 g, 50 mmol) was dissolved in deionized water and made up to 100 ml to give a 0.5-M potassium chloride stock solution. CH 3 COOK (9.8 g, 100 mmol) was dissolved in deionized water and made up to 100 ml to give a 1.0-M potassium acetate stock solution. The original 0.14 M [Mo 2 O 2 S 2 ] 2+ solution was diluted by half to obtain finally a 0.07-M stock solution. Pump system The pump system set up designed by us comprising seven programmable syringe three-way solenoid valve pumps (C3000 model, Tricontinent), whose pumps P1–P6 fitted with a 5-ml syringe and pump P7 fitted with a 12.5-ml syringe. The reactor system was made of a manifold, which was of radial eight-port 1/8-inch design made of polyester, and a tubing extension 4.98 metres long of relatively wide bore (1.6 mm internal diameter) was connected to one of the ports of the mixing manifold to allow dissolution of reagents and conduction of CO 2 gas formation during the reaction. A LabVIEW-based PC interface was used to control the pumps by sending pre-designed stream commands from value matrices in TXT files ( Supplementary Fig. 1 ). At the start of the experiments ( t =0) the total flow rate is set at 4 ml min −1 for all the inputs, and a target volume of 10 ml per reaction is set, which takes 2.5 min per reaction. Including all possible combinations (50 reactions+50 ‘air plug’ spacing; 3 min each) gives a total reaction time of almost 5 h to scan the parameter space. Moreover, the ratios and concentrations within the scanned parameter space varied in such a way that the obtained pH varied between the values 2–5. Synthesis of compound 1 The following volumes of starting reagents were used to synthesize compound 1 : 1.8 ml (K 2 CO 3 0.35 M), 0.3 ml (KCl 0.5 M), 3.2 ml (C 5 O 5 Na 2 0.1 M) and 4.7 ml ([Mo 2 S 2 O 2 ] 2+ 0.07 M). The pH value of the crystallization solution is 3.1 and the temperature for the reaction was 20 °C. Orange rod-like crystals were obtained by evaporation at room temperature after 4 days. Yield of [N(CH 3 ) 4 ]K[(Mo V 2 O 2 S 2 ) 5 (OH) 10 (C 5 O 5 )] · 17 H 2 O ( 1 ): 50 mg, 35.5%, based on Mo V . Infrared (KBr disk): [vtilde] =3,187.8 (w), 1,613.2 (w), 1,477.2 (sh), 1,082.8 (w), 955.56 (sh), 657.6 (w), 545.8 (m) cm −1 . Elemental analysis, calcd for C 9 H 56 KMo 10 NO 42 S 10 (%) (Fw. : 2,169.68 g mol −1 ): C: 4.98; H: 2.60; N: 0.65; K: 1.80; Mo: 44.22; Found: C: 5.12; H: 2.12; N: 0.66; K: 1.97; Mo: 46.02. Synthesis of compound 2 The following volumes of starting reagents were used to synthesize compound 2 : 1.7 ml (C 4 O 4 H 2 0.17 M), 1.0 ml (K 2 CO 3 0.35 M), 1.5 ml (Na 2 MoO 4 0.2 M), 1.3 ml (C 5 O 5 Na 2 0.1 M) and 4.5 ml ([Mo 2 S 2 O 2 ] 2+ 0.07 M). The pH value of the crystallization solution is 2.8 and the temperature for the reaction was 20 °C. Red rod-like crystals were obtained by evaporation at room temperature after 5 days. Yield of K 10 [(Mo V 2 O 2 S 2 )(H 2 O) 2 (C 5 O 5 ) 2 ][Mo 12 O 36 (C 4 O 4 ) 4 ] · 14 H 2 O ( 2 ): 20 mg, 1.9%, based on Mo V . Infrared (KBr disk): [vtilde] =3,457.7 (m), 1,627.6 (s), 1,480.1 (sh), 1,090.6 (w), 930.5 (sh), 605.5 (m) cm −1 . Elemental analysis, calcd for C 26 H 32 K 10 Mo 14 O 80 S 2 (%) (Fw. : 3,422.76 g mol −1 ): C: 9.12; H: 0.94; K: 11.42; Mo: 39.24; Found: C: 8.92; H: 0.76; K: 11.24; Mo: 40.66. Synthesis of compound 3 The following volumes of starting reagents were used to synthesize compound 3 : 2.9 ml (C 4 O 4 H 2 0.17 M), 1.4 ml (K 2 CO 3 0.35 M), 1.6 ml (Na 2 MoO 4 0.2 M) and 4.1 ml ([Mo 2 S 2 O 2 ] 2+ 0.07 M). The pH value of the crystallization solution is 3.0 and the temperature for the reaction was 20 °C. Red rod-like crystals were obtained by evaporation at room temperature after 7 weeks. Yield of [N(CH 3 ) 4 ] 4 K 18 [((Mo V 2 O 2 S 2 ) 3 (OH) 4 (C 4 O 4 )) 6 (OH) 2 (Mo 6 O 21 (H 2 O)) 2 ][Mo 12 O 36 (C 4 O 4 ) 4 ] · 79 H 2 O ( 3 ): 35 mg, 22.4%, based on Mo V . Infrared (KBr disk): [vtilde] =3,412.4 (s), 1,625.7 (sh), 1,534.1 (sh), 1,475.3 (s), 1,095.4 (w), 947.8 (sh), 775.2 (m), 592.0 (m), 504.29 (m) cm −1 . Elemental analysis, calcd for C 56 H 236 K 18 Mo 60 N 4 O 261 S 36 (%) (Fw. : 1,2756.88 g mol −1 ): C: 5.27; H: 1.86; N: 0.44; S: 9.05, K: 5.52, Mo: 45.12; Found: C: 5.34; H: 1.74; N: 0.44; S: 8.85, K: 5.59, Mo: 45.70. Synthesis of compound 4 The following volumes of starting reagents were used to synthesize compound 4 : 2.8 ml (C 4 O 4 H 2 0.17 M), 1.9 ml (K 2 CO 3 0.35 M), 0.7 ml (Na 2 MoO 4 0.2 M), 0.3 ml (KCl 0.5 M) and 4.3 ml ([Mo 2 S 2 O 2 ] 2+ 0.07 M). The pH value of the crystallization solution is 3.0 and the temperature for the reaction was 20 °C. Red sheet crystals were obtained by evaporation at room temperature after 6 weeks. Yield of [N(CH 3 ) 4 ] 3 K 11.5 Na 0.5 I[((Mo V 2 O 2 S 2 ) 3 (OH) 4 (C 4 O 4 )) 6 (OH) 2 (Mo 6 O 21 (H 2 O)) 2 ] · 19 H 2 O: 25 mg, 18.9%, based on Mo V . Infrared (KBr disk, [vtilde] =3,411.5 (m), 1,625.7 (m), 1,535.1 (sh), 1,477.2 (s), 1,095.4 (w), 948.8 (sh), 866.8 (w), 776.2 (m), 590.1 (w), 506.2 (w) cm −1 . Elemental analysis, calcd for C 36 H 104 IK 11.5 Mo 48 N 3 Na 0.5 O 149 S 36 (%) (Fw. : 9,310.67 g mol −1 ): C: 4.64; H: 1.13; N: 0.45; S: 12.40; K: 4.83; Na: 0.12; Mo: 49.46; Found: C: 4.42, H: 1.09, N: 0.31, S: 12.67, K: 4.97, Na: 0.14, Mo: 50.55 (about 71 lattice water molecules were lost compared with X-ray crystallographic data, 4 ). Synthesis of compound 5 The following volumes of starting reagents were used to synthesize compound 5 : 1.9 ml (C 4 O 4 H 2 0.17 M), 2.5 ml (K 2 CO 3 0.35 M), 0.9 ml (Na 2 MoO 4 0.2 M), 1.0 ml (KAc 1.0 M) and 3.7 ml ([Mo 2 S 2 O 2 ] 2+ 0.07 M). The pH value of the crystallization solution is 4.6 and the temperature for the reaction was 20 °C. Orange block crystals were obtained by evaporation at room temperature after 4–5 weeks. Yield of K 14 [((Mo V 2 O 2 S 2 ) 3 (OH) 4 (C 4 O 4 )) 4 (Mo 5 O 18 (CH 3 COO)) 2 ] · 52 H 2 O ( 5 ): 10 mg, 6.3%, based on Mo V . Elemental analysis, calcd for C 20 H 126 K 14 Mo 34 O 148 S 24 (%) (Fw. : 7,314.05 g mol −1 ): C: 3.28; H: 1.74; S: 10.52, K: 7.48, Mo: 44.59; Found: C: 3.36; H: 2.00; S: 10.62, K: 7.22, Mo: 44.66. Infrared (KBr disk): [vtilde] =3,417.2 (s), 2,925.5 (w), 1,623.8 (s), 1,515.8 (sh), 1,103.1 (w), 941.1 (sh), 871.7(m), 758.9 (m), 662.4 (m), 498.5 (m) cm −1 . Synthesis of compound 6 The following volumes of starting reagents were used to synthesize compound 5 : 2.7 ml (C 4 O 4 H 2 0.17 M), 4.0 ml (K 2 CO 3 0.35 M), 0.5 ml (KCl 0.5 M), 2 ml DMF and 0.8 ml ([Mo 2 S 2 O 2 ] 2+ 0.07 M). The pH value of the crystallization solution is 3.2 and the temperature for the reaction was 20 °C. Light orange crystals obtained by evaporation at room temperature within 10 days giving ( 6 ) as [N(CH 3 ) 4 ] 4 K 8 [((Mo V 2 O 2 S 2 ) 3 (OH) 4 (C 4 O 4 )) 3 (C 4 O 4 ) 6 (N(CH 3 ) 2 CHO) 3 ] · 30 H 2 O: The yield is low but reproducible 1 mg, 3.1%, based on Mo V . Elemental Analysis, calcd for C 61 H 141 N 7 S 18 O 99 K 8 Mo 18 (%) (Fw. : 5,173.65 g mol −1 ): C: 14.16; H: 2.75; N: 1.90 S: 11.16, K: 6.05, Mo: 33.38; Found: C: 13.81; H: 2.58; N: 1.85; K: 5.95; Mo: 33.15. Infrared (KBr, cm −1 ): [vtilde] =3,425.9 (m), 1,787.7 (w), 1,655.6 (sh), 1,509.9 cm −1 . FT–IR spectroscopy The materials were prepared as KBr pellets and Fourier transform–infrared spectra were collected in transmission mode using a JASCO FT-Infrared-410 spectrometer or a JASCO FT-Infrared 4100 spectrometer. Characteristic Infrared bands are given for compounds 1 – 6 in cm −1 ; intensities denoted as s=strong, m=medium, w=weak, sh=sharp ( Supplementary Figs 12–17 ). Ultraviolet–visible spectroscopy Ultraviolet–visible spectra were collected for compounds 1 – 4 using a JASCO V-670 spectrometer in the solution in absorption mode within the wavelength range 200–500 nm ( Supplementary Figs 18–21 ). Thermogravimetric analysis Thermogravimetric analysis was performed on a TA Q500 instrument from room temperature to 1,000 °C at a heating rate of 5 °C per min in a N 2 atmosphere ( Supplementary Figs 22–27 ). Mass spectrometry Electrospray-ionization mass spectrometry (ESI-MS) was performed using a Bruker microTOF-Q quadrupole time-of-flight mass spectrometer. The mass spectrum of the compound 1 {Mo 10 (C 5 )} was measured in acetonitrile ( Supplementary Table 3 ) and compounds 3 {Mo 60 } ( Supplementary Table 4 ) and 4 {Mo 48 } ( Supplementary Table 5 ) were conducted in a mixture of deionized water and acetonitrile (5:95%). X-ray structure analysis Single-crystal X-ray data were collected at 150 K on a Bruker APEX2 CCD diffractometer using graphite monochromated MoK α radiation ( λ =0.71069 Å). The linear absorption coefficients, scattering factors for the atoms and anomalous dispersion corrections were taken from the International Tables for X-ray crystallography. Data integration and reduction were processed with Apex2 software package (SAINT & SADABS). An empirical absorption correction was applied to the collected reflections with SADABS to correct incident and diffracted beam absorption effects. The structure was solved by the direct method using SHELXS-97 and was refined on F 2 by the full-matrix least-squares technique using the SHELXL-97 (refs 32 , 33 ) programme package of WINGX [34] . It is important to note that with compounds {Mo 34 }, {Mo 48 } and {Mo 60 }, we are moving outside the realm of small molecule crystallography and are dealing with refinements and problems that lie between small molecule and protein crystallography. As a result, we cannot expect refinements and statistics to follow the path of crystals with much smaller unit cells. The lattice parameters and structural data are collected in Supplementary Table 6 , see also Supplementary Data 1–6 . Accession codes: The X-ray crystallographic coordinates for structures reported in this Article have been deposited at the Cambridge Crystallographic Data Centre (CCDC), under deposition number CCDC 936796, 936799, 936798, 936797, 975305 and 975304. These data can be obtained free of charge from The Cambridge Crystallographic Data Centre via www.ccdc.cam.ac.uk/data_request/cif . How to cite this article : Zang, H.-Y. et al. Discovery of gigantic molecular nanostructures using a flow reaction array as a search engine. Nat. Commun. 5:3715 doi: 10.1038/ncomms4715 (2014).